MBNL1 and RBFOX2 cooperate to establish a splicing programme involved in pluripotent stem cell differentiation Reprogramming somatic cells into induced pluripotent stem cells (iPSCs) has provided huge insight into the pathways, mechanisms and transcription factors that control differentiation. Here we use high-throughput RT–PCR technology to take a snapshot of splicing changes in the full spectrum of high- and low-expressed genes during induction of fibroblasts, from several donors, into iPSCs and their subsequent redifferentiation. We uncover a programme of concerted alternative splicing changes involved in late mesoderm differentiation and controlled by key splicing regulators MBNL1 and RBFOX2. These critical splicing adjustments arise early in vertebrate evolution and remain fixed in at least 10 genes (including PLOD2, CLSTN1, ATP2A1, PALM, ITGA6, KIF13A, FMNL3, PPIP5K1, MARK2 and FNIP1), implying that vertebrates require alternative splicing to fully implement the instructions of transcriptional control networks. Intense efforts are dedicated to the study of stem cells because of the potential medical benefits and the insights into differentiation that they offer [1] , [2] , [3] , [4] . Pluripotent stem cells can be induced into ectoderm, endoderm and mesoderm, recapitulating the early events in embryogenesis [5] , [6] . Early differentiation involves the induction of cell line-specific transcription factors, whereas the late stages of differentiation are less well characterized [4] , [7] , [8] , [9] . Alternative splicing is a means by which the genome can control the expression of different protein isoforms that can drive fundamental cellular changes and this is mostly achieved through the differential expression of RNA-binding proteins [10] , [11] , [12] . Ever since the discovery that alternative splicing controls Drosophila sex differentiation over 20 years ago, alternative splicing has been suggested to be a potential mechanism whereby different protein isoforms could be delivered to implement mammalian differentiation [13] , [14] , [15] , [16] . Several studies have also hinted at an involvement of alternative splicing in pluripotency and pluripotent stem cell differentiation along various pathways [17] , [18] . For example, different isoforms of the forkhead transcription factor Foxp1 have differential effects on the induction of key pluripotency genes such as Oct4 and Nanog [19] . Similarly, alternative splice forms of DNMT3B are specific to stem cells, implying that layered and integrated regulation of gene expression occurs at the levels of transcription and splicing [20] . Current analyses of genome-wide changes in alternative splicing rely mostly on two techniques: microarrays and next-generation sequencing. However, these techniques are heavily biased towards the most highly expressed genes and cannot quantify alternative splicing of medium- and low-expressed genes that can be expressed at 10,000 times lower levels than housekeeping genes [21] . We recently developed a unique high-throughput RT–PCR platform to probe the entire repertoire of over 3,000 alternative splice events annotated in the RefSeq database without bias against medium- and low-expressed genes [22] , and further used this technique to probe the involvement of 81 different RNA-binding proteins in epithelial-to-mesenchymal transition by comparing the splicing profiles of epithelial and mesenchymal tissues with those of the cells lines treated with siRNAs against the 81 proteins [23] . Here we have used high-throughput RT–PCR to implicate the RNA-binding protein Muscleblind (MBNL1) in differentiation of stem cells, and we show that essential induction of MBNL1 late during mesoderm differentiation controls a splicing programme that induces and represses specific exons at the RNA level. Alternative splicing programs in fibroblasts and stem cells To analyse the programme of alternative splicing changes occurring in human pluripotent stem cells during stem cell induction, maintenance and differentiation, we designed a large-scale screening strategy. Using high-throughput PCR, we previously screened the entire NCBI Reference Sequence (RefSeq) database for the presence or absence of both of two predicted isoforms at thousands of loci. From these, detected, alternatively spliced events we selected 303 high-quality PCRs from across the alternative exons, using only purity and yield of the two PCR products in 10 different cell lines as parameters We used these high-quality PCRs to study alternative splicing in pluripotent stem cells in more detail because they occur in an essentially random and functionally diverse cross-section of genes [22] . Alternative splicing was studied in human skin fibroblasts and their induced pluripotent stem cells (iPSCs) and then also in fibroblasts redifferentiated from those iPSCs [24] . We observed a reversible programme of alternative splicing ( Fig. 1a correlation R =−0.88). Equally remarkably, the inclusion levels of 15 of the 303 alternative exons shifted >50 percentage points on average between pluripotent stem cells and their parental and daughter fibroblasts (and >40% in both transitions Supplementary Data 1 ). Such extreme shifts in alternative splicing are rarely described and are defined as ‘switch-like’ [25] , [26] , [27] . Thus, using a randomly selected set of alternative splicing events we have uncovered an unprecedented programme of reversible regulated switch-like alternative splicing in stem cells, whereby 5% of a functionally random snapshot of all alternative splicing events can be induced to shift reversibly from predominantly one isoform to nearly exclusively the other, between the fibroblastic and pluripotent states. Furthermore, there is a very good correlation ( R =0.824, Supplementary Fig. S2 ) between percent-spliced-in values obtained with RNA-Seq data [28] and our PCR-based methodology for those events in which RNA-seq data had enough read depth to produce confident PSI estimates (104 out of 303 mapped events; Supplementary Data 1 ). To establish if these alternative splicing changes were a general feature of stem cells we performed manual end-point PCRs with the 15 switch-like splicing events on three different pluripotent stem cells and their resulting differentiated and parental fibroblasts. Samples included the well-characterized H9 embryonic stem cells and their redifferentiated fibroblasts. In all cases we observed a near complete and fully reversible shift from one isoform to the other between stem cells and fibroblasts ( Fig. 1b ). 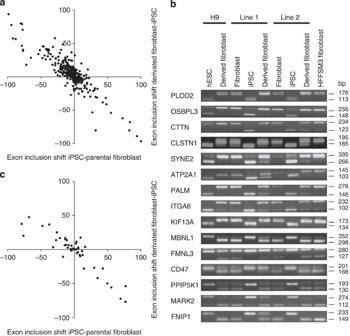Figure 1: A reversible splicing programme in pluripotent stem cells. (a) Scatter plot showing reversible splicing changes in 303 exons in a diverse array of genes. PCRs were performed on cDNA from parental fibroblasts, their induced pluripotent stem cells (iPSCs) and from re-differentiated fibroblasts from these iPSCs. The transitions in splicing are shown on thexaxis (iPSCs-parental fibroblasts) andyaxis (re-differentiated fibroblasts-iPSCs) respectively. (b) 15 switch-like splicing changes from (a) were assessed in the various fibroblast–to-stem cell transitions indicated. The upper and lower bands on each gel represent the long (exon-included) and short (exon-omitted) isoforms respectively. Full gel scans are shown inSupplementary Fig. 6. (c) The panel of 47 splice events from23were also assayed for their splicing switches as in (a) to test their appropriateness for studying the splicing factors that control differentiation. Figure 1: A reversible splicing programme in pluripotent stem cells. ( a ) Scatter plot showing reversible splicing changes in 303 exons in a diverse array of genes. PCRs were performed on cDNA from parental fibroblasts, their induced pluripotent stem cells (iPSCs) and from re-differentiated fibroblasts from these iPSCs. The transitions in splicing are shown on the x axis (iPSCs-parental fibroblasts) and y axis (re-differentiated fibroblasts-iPSCs) respectively. ( b ) 15 switch-like splicing changes from ( a ) were assessed in the various fibroblast–to-stem cell transitions indicated. The upper and lower bands on each gel represent the long (exon-included) and short (exon-omitted) isoforms respectively. Full gel scans are shown in Supplementary Fig. 6 . ( c ) The panel of 47 splice events from [23] were also assayed for their splicing switches as in ( a ) to test their appropriateness for studying the splicing factors that control differentiation. Full size image Modulation of alternative splicing programs To create a tool to understand the systems biology of splicing, we recently knocked down 81 potential splicing factors in various cell lines and performed RT–PCRs across 47 alternatively spliced regions in different genes [23] . Here we monitored these 47 splicing events using RNA extracted from iPSCs and their parental fibroblasts [24] with the aim of identifying the splicing factors involved in pluripotency and reprogramming ( Supplementary Data 2 ). The splicing profile of these 47 PCRs showed an equivalent near-perfect anti-correlation of R =−0.91 in reversible stem cell induction and redifferentiation, demonstrating that this smaller set of 47 alternative splice events can be used to investigate the splicing control mechanisms involved in stemness and maintenance of pluripotency ( Fig. 1c ). The differences in percent-spliced-in values, in these 47 alternative splice events, induced in pluripotency (iPSC values-original fibroblasts) were then compared with the differences induced when we knocked down 81 splicing potential factors (knockdown-control, Supplementary Data 3 and 4 ). Strikingly, the profile of MBNL1 knockdown correlated most strongly ( R =0.6) with the splicing profile of the induction of pluripotency ( Fig. 2a , lines 1 and 2). 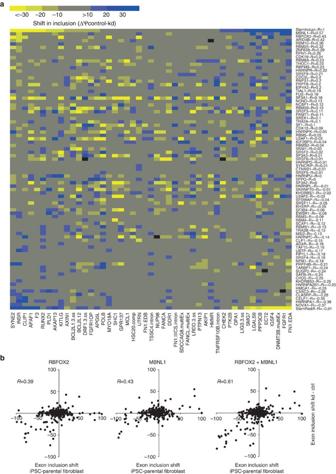Figure 2: Implication of RBFOX2 and MBNL1 splicing factors in pluripotent stem cell induction. (a) Heat map showing percent-spliced-in shifts for the 47 alternate splicing events (xaxis) between fibroblasts and iPSCs and when 81 different knockdowns were performed in two to five cell lines23. The splicing factors are ordered according to the Pearson correlation (R) of their splicing profiles (k.d.—control,yaxis) with that of pluripotent stem cell induction (iPSC—parental fibroblast,xaxis) on the first line. (b) Scatter plots comparing splicing changes for the 303 exons in pluripotent stem cell induction with RBFOX2, MBNL1 and the double-knockdown (RBFOX2 and MBNL1) in HFFSM3 fibroblasts. Pearson correlations (R values) are shown. Figure 2: Implication of RBFOX2 and MBNL1 splicing factors in pluripotent stem cell induction. ( a ) Heat map showing percent-spliced-in shifts for the 47 alternate splicing events ( x axis) between fibroblasts and iPSCs and when 81 different knockdowns were performed in two to five cell lines [23] . The splicing factors are ordered according to the Pearson correlation ( R ) of their splicing profiles (k.d.—control, y axis) with that of pluripotent stem cell induction (iPSC—parental fibroblast, x axis) on the first line. ( b ) Scatter plots comparing splicing changes for the 303 exons in pluripotent stem cell induction with RBFOX2, MBNL1 and the double-knockdown (RBFOX2 and MBNL1) in HFFSM3 fibroblasts. Pearson correlations (R values) are shown. Full size image MBNL1 is a key gene involved in the myotonic dystrophies, DM1 and DM2, which were the first defined RNA diseases. One normal function of Muscleblind is to modulate splicing during muscle and heart development [29] , [30] , [31] , [32] , [33] , [34] . The second most correlated knockdown was RBFOX2, which is a well-characterized splicing factor that we and others have implicated in epithelial-to-mesenchymal transition and invasion [22] , [23] , [34] , [35] . To confirm the association of these two proteins with stem cell differentiation, we knocked down MBNL1 and RBFOX2 in fibroblasts, alone or in combination, and performed automated RT–PCR for the 303 original alternative splicing events. We observed a significant correlation of splicing changes between individual MBNL1 and RBFOX2 knockdowns and the changes occurring upon induction of the original fibroblasts into the pluripotent state ( R =0.4). Remarkably, the correlation was even higher ( R =0.6) between splicing changes associated with pluripotent stem cell derivation and those occurring in fibroblasts and a double-knockdown of MBNL1 and RBFOX2 ( Fig. 2b ). Manual PCR for the 15 switch-like splice events further confirmed these results, with five of the exons (PLOD2, OSBPL3, CTTN, CLSTN and SYNE2) strongly enhanced by RBFOX2 (that is, inclusion of these exons was strongly inhibited by knockdown of RBFOX2), whereas the remaining 10 exons were either enhanced or inhibited by MBNL1 ( Fig. 3a,b ). 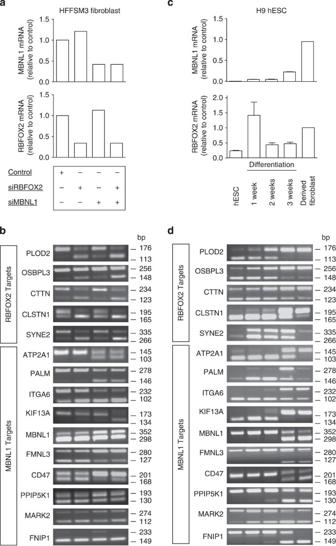Figure 3: The stem cell splicing programme is controlled by RBFOX2 and MBNL1 respectively after commitment. (a) Bar graphs showing MBNL1 and RBFOX2 expression levels in HFFSM3 fibroblasts used, assessed by qPCR. Fibroblasts were transfected by siRNA pool (one ‘ON-TARGET plus smartpool’ equivalent to four siRNAs per gene). We used scrambled siRNA as negative control. (b) Agarose gel showing change in splicing of the 15 targets in HFFSM3 fibroblasts knocked down for RBFOX2 or MBNL1. Full gel scans are shown inSupplementary Fig. S6. (c) Bar graphs showing RBFOX2 and MBNL1 expression levels in H9 hESCs following induction of redifferentiation, assessed by qPCR. Shown are the results of two independent experiments performed in triplicate. Error bars show the range. (d) Time course of splicing changes during H9 hESC-fibroblast differentiation. The agarose gel shows an early and gradual shift in splicing of the five RBFOX2 targets (first five lines) and a later and more sudden switch in splicing around half way through the differentiation protocol for the MBNL1 targets (remaining lines). Figure 3: The stem cell splicing programme is controlled by RBFOX2 and MBNL1 respectively after commitment. ( a ) Bar graphs showing MBNL1 and RBFOX2 expression levels in HFFSM3 fibroblasts used, assessed by qPCR. Fibroblasts were transfected by siRNA pool (one ‘ON-TARGET plus smartpool’ equivalent to four siRNAs per gene). We used scrambled siRNA as negative control. ( b ) Agarose gel showing change in splicing of the 15 targets in HFFSM3 fibroblasts knocked down for RBFOX2 or MBNL1. Full gel scans are shown in Supplementary Fig. S6 . ( c ) Bar graphs showing RBFOX2 and MBNL1 expression levels in H9 hESCs following induction of redifferentiation, assessed by qPCR. Shown are the results of two independent experiments performed in triplicate. Error bars show the range. ( d ) Time course of splicing changes during H9 hESC-fibroblast differentiation. The agarose gel shows an early and gradual shift in splicing of the five RBFOX2 targets (first five lines) and a later and more sudden switch in splicing around half way through the differentiation protocol for the MBNL1 targets (remaining lines). Full size image Control of alternative splicing programs by MBNL1 and RBFOX2 One of the major questions in developmental biology is to understand the events related to the specification of the different cell lineages in the embryo. As pluripotent stem cell differentiation is considered to occur in two phases (before and after commitment) [4] , we sought to establish whether our splicing programme was associated with specification to committed stem cells or to the subsequent differentiation step. We studied alternative splicing of the 15 switch-like targets in H9 human embryonic stem cells (hESCs) that differentiated into early ectoderm, endoderm and mesoderm precursors and surprisingly found only very minor changes in alternative splicing of the 5 RBFOX2-controlled exons (first 5 lines of Supplementary Fig. S1a ) and no change at all for the 10 MBNL1-controlled exons. We confirmed that the pluripotent stem cells had indeed committed to the three germ layers using two marker genes for each type ( Supplementary Fig. S1b , primers listed in Supplementary Table S1 ). To confirm that the MBNL- and RBFOX-controlled splicing programme was a late event in differentiation we took samples of stem cells at 1, 2 and 3 weeks into the 5-week differentiation protocol. qPCR analysis demonstrated an early upregulation of RBFOX2 and a later upregulation of MBNL1 ( Fig. 3c ). Consistent with this, manual end-point PCR demonstrated a gradual change in the five RBFOX2 targets, starting in the first week of differentiation, whereas the 10 MBNL1 targets changed later and more sharply, mostly between 2–3 weeks of differentiation ( Fig. 3d ). Changes in splicing were essentially complete after 3 weeks of differentiation consistent with those changes occurring during the later stages of mesoderm differentiation. Next we checked whether MBNL1 and RBFOX2 were indeed downregulated in pluripotent stem cells and we observed almost complete abrogation of MBNL1 expression and significant downregulation of RBFOX2 at both the RNA and protein levels in all stem cell types, irrespective of their provenance ( Fig. 4 ; primers listed in Supplementary Table S1 ). Downregulation of MBNL and RBFOX genes was also confirmed by retrospective analysis of our previously published microarray data for all three MBNL and RBFOX orthologues [24] . Both MBNL1 and MBNL2 mRNAs were downregulated in pluripotent stem cells with MBNL1 being the more abundant in fibroblasts, whereas RBFOX2 was essentially the only RBFOX gene present in these cell types ( Supplementary Fig. S3a ). We also confirmed upregulation of the fibroblast-specific exons of the RBFOX2-enhanced exon of PLOD2 and the MBNL1-enhanced exon of PALM by raising specific antibodies against the alternatively spliced peptides ( Supplementary Fig. S3b ). We conclude that committed stem cells undergo a massive reversible reprogramming of splicing from inclusion or exclusion of exons to the opposite splice isoform during differentiation (>5% of exons assayed) and that the Muscleblind and Fox proteins (mostly MBNL1 and RBFOX2) control the vast majority of this programme. 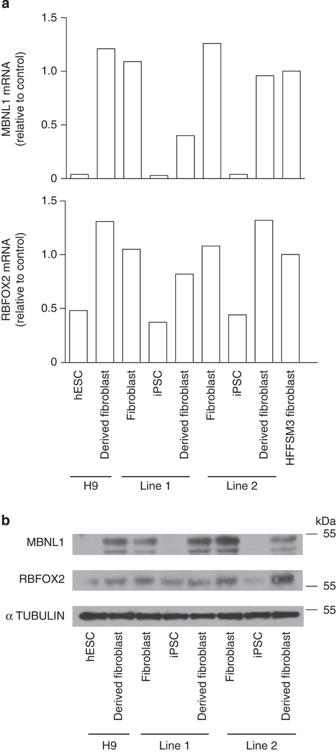Figure 4: Upregulation of RBFOX2 and MBNL1 expression after commitment. (a) Bar graphs showing the expression level of MBNL1 and RBFOX2 in parental fibroblasts, corresponding iPSCs, H9 hESCs and fibroblast-differentiated cells (samples fromFig. 1b) assessed by qPCR. (b) Western blots showing global expression of MBNL1 and RBFOX2. Uncropped images of blots are shown inSupplementary Fig. S7. Figure 4: Upregulation of RBFOX2 and MBNL1 expression after commitment. ( a ) Bar graphs showing the expression level of MBNL1 and RBFOX2 in parental fibroblasts, corresponding iPSCs, H9 hESCs and fibroblast-differentiated cells (samples from Fig. 1b ) assessed by qPCR. ( b ) Western blots showing global expression of MBNL1 and RBFOX2. Uncropped images of blots are shown in Supplementary Fig. S7 . Full size image MBNL1 and RBFOX2 alternative splicing programs are conserved To confirm the specificity of alternative splicing changes for late mesoderm differentiation we compared splicing changes for the 15 genes in mouse and human stem cells that we fully differentiated into late ectoderm, endoderm and mesoderm [5] . In this case we noted that 12 of the alternative splicing events (all excluding OSBPL3, CTTN and CD47) shifted in human and mouse mesoderm and very few of these events changed in ectoderm or endoderm ( Fig. 5 ). Control markers for ectoderm, endoderm and mesoderm differentiation were verified by qPCR ( Supplementary Fig. S4 ). We conclude that these 12 alternative splice events undergo a conserved programme that qualitatively regulates mesodermal gene expression. These results led us to suspect that co-regulation of MBNL1 and RBFOX2 was necessary for the pluripotent stem cell splicing signature and for their differentiation. To test this we inhibited their re-expression in pluripotent stem cells after 2 weeks of redifferentiation. Although we did not observe any effect on the expression of specific markers of pluripotency OCT4, NANOG and SOX2 ( Supplementary Fig. S5a ), we confirmed that splicing changes occurring late during differentiation can be reversed, either by individual knockdown of RBFOX2 and MBNL1 or by double-knockdown of both splicing factors ( Fig. 6 ). The knockdowns in these samples were consistent with an early induction of RBFOX2 and a late induction of MBNL1. 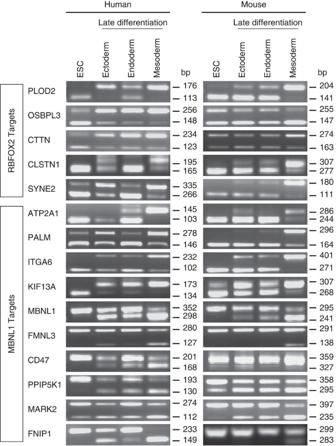Figure 5: Conservation of specificity of mesoderm-specific splicing in mammals. Agarose gels showing the alternative splicing of the 15 alternative splicing events identified inFig. 3during human and mouse stem cell differentiation into the three germ cell layers. Upper and lower bands represent the long and short isoforms respectively. Full gel scans are shown inSupplementary Fig. S6. Figure 5: Conservation of specificity of mesoderm-specific splicing in mammals. Agarose gels showing the alternative splicing of the 15 alternative splicing events identified in Fig. 3 during human and mouse stem cell differentiation into the three germ cell layers. Upper and lower bands represent the long and short isoforms respectively. Full gel scans are shown in Supplementary Fig. S6 . 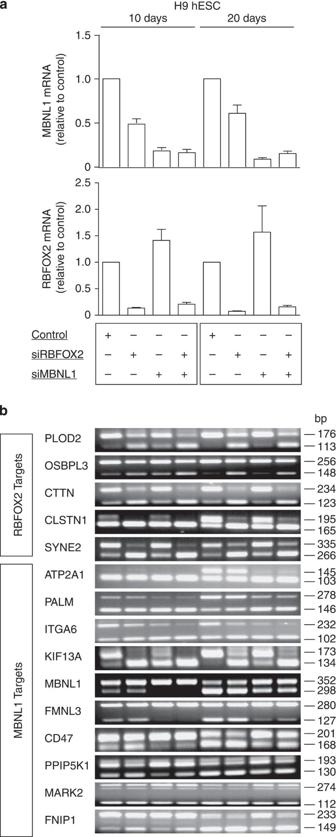Figure 6: Reversal of fibroblast splicing profile by inhibition of RBFOX2 and MBNL1 re-expression. (a) Bar graphs showing the knockdown efficiency of RBFOX2 and MBNL1 in differentiating H9 hESCs at two different time points, assessed by qPCR. Two treatments of siRNA pool (one ‘ON-TARGET plus smartpool’ equivalent to 4 siRNAs per gene) were applied at 2-day intervals before harvesting cells. The left hand and right hand side represent siRNA pool applications commencing at either 7 or at 15 days after launching the differentiation. We used scrambled RNA as negative control. Shown are means and s.d. of three independent experiments performed in triplicate. (b) RT-PCRs for the 15 switch-like exons were studied in the differentiating H9 hESCs knocked down for RBFOX2 (siRBFOX2), MBNL1 (siMBNL1) or both. Full gel scans are shown inSupplementary Fig. S6. Full size image Figure 6: Reversal of fibroblast splicing profile by inhibition of RBFOX2 and MBNL1 re-expression. ( a ) Bar graphs showing the knockdown efficiency of RBFOX2 and MBNL1 in differentiating H9 hESCs at two different time points, assessed by qPCR. Two treatments of siRNA pool (one ‘ON-TARGET plus smartpool’ equivalent to 4 siRNAs per gene) were applied at 2-day intervals before harvesting cells. The left hand and right hand side represent siRNA pool applications commencing at either 7 or at 15 days after launching the differentiation. We used scrambled RNA as negative control. Shown are means and s.d. of three independent experiments performed in triplicate. ( b ) RT-PCRs for the 15 switch-like exons were studied in the differentiating H9 hESCs knocked down for RBFOX2 (siRBFOX2), MBNL1 (siMBNL1) or both. Full gel scans are shown in Supplementary Fig. S6 . Full size image Examination of the potential physiological roles of the 12 switch-like exons in mammalian mesoderm revealed that nearly all of them encode parts of proteins involved in membrane dynamics, cell adhesion, migration and polarity ( Fig. 7a ). To support the notion that the observed alternative isoforms have important roles in controlling cellular morphology, we examined their conservation further across evolution. All the genes probably fulfil generic cell functions as they were already present in early metazoans or coelomates. Equally strikingly we found that 8 of the 12 alternatively spliced exons arose concurrently with gene duplications, mostly between jawless and jawed vertebrates ( Fig. 7a ). For the majority of genes, we found the presence of alternative exons associated with alternative splicing after duplications, whereas no exon homologue could be detected before duplications, suggesting that exon gain and alternative splicing were innovative features selected together to control development in jawed vertebrates. Similar findings on exonic splicing elements and duplications were drawn from genome-wide studies [36] . Consistent with the function of these conserved splicing events in membrane dynamics, cell adhesion, migration and polarity, we observed a halving of cell size when either MBNL1 or RBFOX2 re-expression was inhibited during stem cell redifferentiation, countering the normal growth in cell size during differentiation ( Fig. 7b ). Cells had less stress fibres with more actin bundles ( Supplementary Fig. S5b ). Cells also had reduced level of N-CADHERIN and interestingly increased level of E-CADHERIN, an epithelial marker ( Fig. 7c ). Consistent with E-CADHERIN re-expression, the RBFOX2 and MBNL1 knockdowns trigger a reduction of the transcription factor TWIST, which represses the expression of E-CADHERIN [37] ( Supplementary Fig. S5c ). We conclude therefore that cooperation between MBNL1 and RBFOX2 is essential for committed stem cell differentiation. 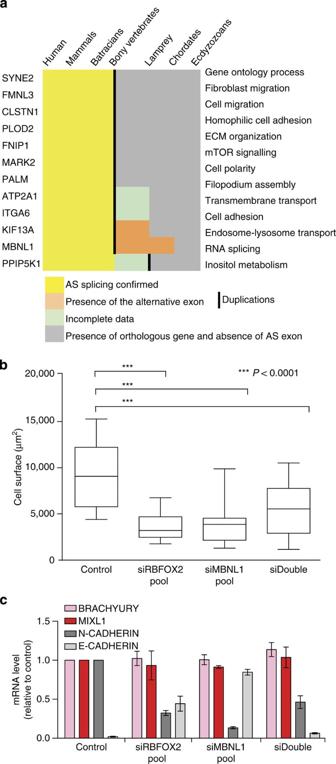Figure 7: Alternative splicing of RBFOX2/MBNL1 target genes is conserved in teleostomes and is required for fibroblast differentiation. (a) Metazoan genomes deposited in Ensembl were searched for orthologs and paralogs of each target gene and for the presence (yellow) or absence (grey) of potential AS exons (Accession numbers inSupplementary Table S2). Yellow indicates that alternatively spliced mRNAs were detected in EST databases (orange indicates that EST number was too low to conclude). Green indicates missing genomic and EST data. Duplications are indicated by thick lines. (b) H9 hESCs were differentiated for 2 weeks and then treated twice every 2 days with an siRNA pool against RBFOX2, MBNL1 or both (siDouble). We used scrambled RNA as negative control (Control). Cells were stained with phalloidin (anti-actin) and Hoechst stain was used for nuclear staining to quantify the effect of RBFOX2 and/or MBNL1 silencing on hESC-derived fibroblast morphology. Box-plots show the average area of 33 cells for each condition. Whiskers correspond to the 5–95 percentiles, boxes, to the 25–75 percentiles and the band inside the box, to the median. Statistical analysis was performed using an unpairedt-test (***P<0.0001,n=2). (c) Bar graph showing the expression levels of differentiation markers BRACHYURY, MIXL1, N-CADHERIN and E-CADHERIN in H9 hESCs after the knockdowns at 2 weeks into the fibroblast differentiation, assessed by qPCR. Shown are the results of two independent experiments performed in triplicate. Error bars show the range. Figure 7: Alternative splicing of RBFOX2/MBNL1 target genes is conserved in teleostomes and is required for fibroblast differentiation. ( a ) Metazoan genomes deposited in Ensembl were searched for orthologs and paralogs of each target gene and for the presence (yellow) or absence (grey) of potential AS exons (Accession numbers in Supplementary Table S2 ). Yellow indicates that alternatively spliced mRNAs were detected in EST databases (orange indicates that EST number was too low to conclude). Green indicates missing genomic and EST data. Duplications are indicated by thick lines. ( b ) H9 hESCs were differentiated for 2 weeks and then treated twice every 2 days with an siRNA pool against RBFOX2, MBNL1 or both (siDouble). We used scrambled RNA as negative control (Control). Cells were stained with phalloidin (anti-actin) and Hoechst stain was used for nuclear staining to quantify the effect of RBFOX2 and/or MBNL1 silencing on hESC-derived fibroblast morphology. Box-plots show the average area of 33 cells for each condition. Whiskers correspond to the 5–95 percentiles, boxes, to the 25–75 percentiles and the band inside the box, to the median. Statistical analysis was performed using an unpaired t -test (*** P <0.0001, n =2). ( c ) Bar graph showing the expression levels of differentiation markers BRACHYURY, MIXL1, N-CADHERIN and E-CADHERIN in H9 hESCs after the knockdowns at 2 weeks into the fibroblast differentiation, assessed by qPCR. Shown are the results of two independent experiments performed in triplicate. Error bars show the range. Full size image Gene expression programs are known to change during germ cell differentiation. In this study we implicated a programme of genetic changes, which occur at the level of alternative splicing of genes that is essential for differentiation into one of the primary gene layers. The genes concerned are involved in important cellular functions including membrane dynamics, cell adhesion, migration and polarity ( Fig. 7a ). Of the stem cell switch-like targets we identified, several are also involved in diseases, which the isoforms described here likely impact. MBNL1 itself is responsible for muscular dystrophy, SYNE2 and ATP2A1 are involved in the muscle diseases Emery–Dreyfuss muscular dystrophy (OMIM 612999) and Brody myopathy (OMIM 601003) respectively, ITGA6 is implicated in epidermolysis bullosa junctionalis (OMIM 226730) and PLOD2 is involved in Bruck syndrome (OMIM 609220). Most of the target genes described here are novel targets of the MBNL1 splicing factor. Exceptions include ATP2A1 exon 22 splicing, which was previously shown to be controlled by MBNL1 (refs 38 , 39 ), as was the auto-regulation of MBNL1 exon 5 (ref. 40 ). The high-throughput PCR method we used identifies many robust splicing shifts starting from all the alternative splice events in the highly curated NCBI Reference Sequence database [41] . As the PCR method used (35 cycles) amplifies all expressed genes, even low- and medium-expressed ones, in the precise regions of alternative splicing, it creates lists that are complementary to those generated by RNA-Seq and our findings that stem cell splicing mirrors knockdown of MBNL1 have also been observed by this method [28] . Interestingly, although genes differentially expressed between iPSCs and fibroblasts are enriched in the same physiological pathways [42] , genes regulated at the expression level did not overlap with any of the switch-like target exons identified here. Thus, we propose that regulated splicing cooperates with up- and downregulation of genes [43] to cement the stem cell-induction during reprogramming and differentiation. Both MBNL1 (refs 29 , 44 , 45 ) and RBFOX2 (refs 22 , 46 , 47 ) have been shown to act to enhance exons when they bind downstream and inhibit exons when they bind upstream. Analysis of previously published CLIP-seq data [29] showed that 4 out of 6 (67%) MBNL1 targets identified here with expression in mouse C2C12 cells (MARK2, FMNL3, CD47 and MBNL1 itself) have evidence of MBNL1-binding clusters, either in or directly upstream of the alternative exon, consistent with a role for MBNL1 downregulation in enhancing these exons in stem cells ( Supplementary Data 1 ). It is therefore likely that binding sites for these proteins have been selected soon after duplications, mostly between jawless and jawed vertebrates to control exons important for cell differentiation in vertebrates. In summary, our study reinforces the idea that splicing factors determine the specific nature of a tissue and that the alternative splicing process has been selected during evolution to control the later stages of differentiation following cell cycle control and commitment. Cell culture and in vitro differentiation assays Human neonatal HFFSM3, line 1 and line 2 (ref. 24 ) fibroblasts (kind gift from J.M. Lemaitre, IGF Montpellier, France) were maintained in Dulbecco’s Modified Eagle Medium (DMEM, Life Technologies) containing 10% heat-inactivated fetal bovine serum (FBS, PAA), 2 mM L -Glutamine, 1% penicillin and streptomycin (all from Life Technologies). H9 hESCs (WiCell Research) and iPSCs [24] (kind gift from J.M. Lemaitre, IGF Montpellier, France) were maintained on matrigel (BD Biosciences) with chemically defined mTeSR (Stemcell Technologies) medium. E14 mouse Embryonic Stem Cells (kind gift from T. Bouschet, IGF Montpellier, France) were maintained on feeder-free culture on gelatin (Sigma-Aldrich) with chemically defined ESGRO complete PLUS clonal grade medium (Millipore). In vitro differentiation For the three germ layer differentiation inductions, H9 hESCs were used and differentiated using the protocol described below and in a previous study [5] . Ectoderm model: H9 hESCs were seeded at 300,000 cells per well in six-well plates pre-coated with matrigel (BD Biosciences) with chemically defined mTeSR (Stemcell Technologies) medium for 2 days. From days 3 to 9, H9 cells were cultured in the presence of N2 media (Life Technologies) and specific inhibitor of SMAD pathway, SB431542 (TGFbeta receptor inhibitor) and Noggin (Life Technologies). The medium was changed daily from days 3 to 5 and every 2 days from day 5 to day 9. Endoderm model: H9 hESCs were seeded at 100,000 cells per well in six-well plates pre-coated with matrigel (BD Biosciences) with chemically defined mTeSR (Stemcell Technologies) medium for 1 day. Differentiation was carried out in endoderm priming medium (DMEM 5.5 mM glucose, 10% KO-SR, 2 mM glutamine, 0.1 mM non essential amino-acid, 0,1 mM β-mercaptoethanol) supplemented with Activin A (100 ng ml −1 , Life Technologies), LY296002 (30 μM, Sigma-Aldrish) and FGF2 (10 ng ml −1 , Peprotech) from days 2 to 4, and Wnt3a (25 ng ml −1 , Life Technologies) from days 3 to 4. Then, cells were treated in hepatocyte-priming medium (DMEM 5.5 mM glucose, 2% KO-SR, 2 mM glutamine, 0.1 mM non essential amino-acid, 0,1 mM β-mercaptoethanol), supplemented with BMP4 (50 ng ml −1 , Life Technologies), FGF4 (25 ng ml −1 , Life Technologies) and 1% DMSO from days 5 to 9. Medium was changed daily in both step of differentiation. Mesoderm model: H9 hESCs were seeded at 100,000 cells cm −2 in six-well plates pre-coated with matrigel (BD Biosciences) with chemically defined mTeSR (Stemcell Technologies) medium for 1 day. Cells were cultured in DMEM or F12 medium supplemented with 10% FBS (Hyclone Laboratories), supplemented with VEGF (20 ng ml −1 , Life Technologies). The medium was changed every 2 days. For early differentiation assay, differentiated cells were stopped at 10 days. For late differentiation assay, differentiated cells were re-seeded at 10 days and cultured in the same conditions for 10 more days. For fibroblast differentiation, we used mesoderm model during 3 weeks during which cells were re-seeded once a week. After 3 weeks, VEGF was removed and derivated fibroblasts were cultured as describe above. The same protocols were used for mouse differentiation assays. Knockdown of RBFOX2 and MBNL1 HFFSM3 fibroblasts and fibroblast-differentiated hESC H9 cells were transfected with siRNA ON-TARGET plus SMART pools (Dharmacon, RBFOX2: L-020616-01-0005, MBNL1 L-014136-00-005), and scrambled siRNA (Dharmacon, D-001810-10-05). HFFSM3 fibroblasts were transfected using INTERFERin (Polyplus Transfection). Fibroblast-differentiated H9 cells were transfected twice every 2 days using DharmaFECT (Thermo Scientific). RNA preparation and analysis RNA was isolated from cells using TRI reagent (Sigma-Aldrich). cDNA was generated by reverse transcription with Maxima Reverse Transcriptase (Thermo Scientific). For qPCR assays, gene expression analysis was performed using 5 ng of cDNA and SYBR Green I Master (Roche). mRNA levels were normalized using the mean expression level of GAPDH, RPLO, RPL13A and PBGD. End-point RT–PCR was performed as in ref. 9 . Briefly, reactions were carried out in the Eppendorf Mastercycler PCR Cycler. A first cycle of 15 min at 95 °C was followed by 35 cycles of 30 s at 94 °C, 30 s at 55 °C, and 1 min at 72 °C. The reaction was ended with the extension step of 10 min at 72 °C. Visualization and analysis of amplified products were done using the LabChip HT DNA assay on an automated microfluidic station (Caliper, Hopkinton, MA, USA). For the 15 RBFOX2/MBNL1 selected targets, the amplified products were loaded on 1.5% agarose gel. All primers are detailed in Supplementary Table S1 and Supplementary Data 1 . Immunofluorescence analysis Cells plated on cover slips were fixed for 10 min in 3.7% formalin (in PBS) followed by a 2-min permeabilization with 0.1% Triton X-100 (in PBS) and incubation in PBS containing 0.1% bovine serum albumin. F-actin was revealed using rhodamin-conjugated phalloidin (Sigma-Aldrich) and nuclei were stained using Hoechst 33342 (Sigma-Aldrich). Cells were washed in PBS and water, mounted with DAKO mounting medium and observed under the fluorescence microscope. Cell imaging was performed with a Leica DM6000 (Leica, Wetzlae, Germany) with PL APO grade oil × 20 objective. Images were captured with a Coolsnap HQ2 camera (Roper Scientific Inc.) driven by Metamorph (Molecular Devices) and processed using FiJi software and cell surface area was determined using the measure module of FiJi. Immunoblot analysis For whole-cell extracts, cells were lysed in RIPA buffer or urea buffer depending on the antibody used (RIPA extract for MBNL1, RBFOX2, α-TUBULIN; urea extract for PLOD2, PALM, actin). For RIPA extracts, cells were lysed in RIPA buffer (50 mM Tris–HCl pH 8, 1% ( w / v ) NP-40, 1% ( w / v ) SDS, 0.5% ( w / v ) Na-deoxycholate (DOC), 2 mM EDTA) supplemented with ‘protease inhibitor cocktail’ (Sigma), incubated for 30 min at 4 °C, centrifuged for 30 min at 14,000 g and the protein amounts were quantifed using Bradford method. For urea extracts, cells were lysed in urea buffer (63 mM Tris–HCl pH7.5, 2% ( w / v ) SDS, 5% ( v / v ) 2-mercaptoethanol, 8 M Urea), supplemented with ‘protease inhibitor cocktail’. Cell lysates were next sonicated and centifuged. Supernatants were resolved by SDS–PAGE and transferred to PVDF membranes (Amersham Biosciences). Membranes were blocked in PBS containing 5% ( w / v ) milk powder and 0.05% ( v / v ) Tween-20 (PBST) for 1 h and incubated with primary antibodies at 4 °C overnight. After washing with PBST, membranes were incubated with either anti-mouse or anti-rabbit secondary antibodies conjugated to horseradish peroxidase (HRP) for 1 h at room temperature. Signals were detected with ‘chemiluminescent’ (Thermo Scientific), anti-RBFOX2 (1:100, ab51361, Abcam), anti-MBNL1 (gift from Wolfson Centre for Inherited Neuromuscular Disease MB1a-Mouse Anti-MBNL1 (ref. 48 )), anti-β-actin (1:20,000, AC-74 clone, Sigma), anti-α tubulin (1:15,000, DM1A clone Sigma), anti-mouse IgG-HRP (1:10,000, 0867428, MP Biomedicals) or anti-rabbit IgG-HRP (1:10,000, 0861202, MP Biomedicals). Polyclonal antibodies to human PLOD2 and PALM alternative peptides were generated by CovalAb, Lyon-France by injecting rabbits with synthetic peptides spanning amino acids 446-TLQREKDSPTPETFQMLSPPK-466 and 175-TVEKDKVTGETRVLSST-191, respectively. Antibodies were affinity-purified using a Sepharose bead column conjugated to the relevant peptide. How to cite this article: Venables, J. P. et al . MBNL1 and RBFOX2 cooperate to establish a splicing programme involved in pluripotent stem cell differentiation. Nat. Commun. 4:2480 doi: 10.1038/ncomms3480 (2013).